Small-molecule Bax agonists for cancer therapy Bax, a central death regulator, is required at the decisional stage of apoptosis. We recently identified serine 184 (S184) of Bax as a critical functional switch controlling its proapoptotic activity. Here we used the structural pocket around S184 as a docking site to screen the NCI library of small molecules using the UCSF-DOCK programme suite. Three compounds, small-molecule Bax agonists SMBA1, SMBA2 and SMBA3, induce conformational changes in Bax by blocking S184 phosphorylation, facilitating Bax insertion into mitochondrial membranes and forming Bax oligomers. The latter leads to cytochrome c release and apoptosis in human lung cancer cells, which occurs in a Bax- but not Bak-dependent fashion. SMBA1 potently suppresses lung tumour growth via apoptosis by selectively activating Bax in vivo without significant normal tissue toxicity. Development of Bax agonists as a new class of anticancer drugs offers a strategy for the treatment of lung cancer and other Bax-expressing malignancies. Bax is a major proapoptotic member of the Bcl2 family and a molecule required for cell death that is extensively expressed in both small-cell lung cancer and non-small-cell lung cancer cells [1] , [2] , [3] , suggesting that Bax may be a therapeutic target for lung cancer. Activation of the proapoptotic function of Bax likely occurs through several interdependent mechanisms that involve its translocation from the cytosol to mitochondria [4] , oligomerization and insertion into mitochondrial membranes following cellular stress [5] , [6] , [7] . Previous reports indicate that the proapoptotic activity of Bax can be regulated by phosphorylation, a post-translational modification [2] , [8] , [9] , [10] , [11] . We recently discovered that nicotine-induced Bax phosphorylation at serine 184 (S184) inactivates the proapoptotic function of Bax, leading to increased survival and/or chemoresistance of human lung cancer cells [2] . In contrast, protein phosphatase 2A functions as a physiological Bax phosphatase that not only dephosphorylates Bax at S184 but also potently activates its proapoptotic function [3] . These findings suggest that the S184 phosphorylation site has a key role in regulating the proapoptotic activity of Bax. The three-dimensional (3D) solution structure indicates that the S184 site is located in the hydrophobic C-terminal tail of Bax [12] , which regulates both the subcellular location of Bax and its ability to insert into mitochondrial membranes [2] , [3] , [13] . Mutagenesis analysis reveals that S184 is the major phosphorylation site for functional regulation of Bax activity [14] . Therefore, manipulation of the phosphorylation status of Bax at S184 may represent a novel strategy for cancer treatment. The computational study of molecular recognition is an important strategy for structure-based drug discovery [15] . The DOCK programme suite is composed of sphgen_cpp, grid and DOCK. The programme ‘sphgen_cpp’ generates sets of overlapping spheres that 3D describe the shape of a target pocket [16] . Spheres are initially constructed over the entire surface using the surface representation, and culled to describe only the pocket of interest [15] , [16] . The programme ‘grid’ generates scoring grids derived from the electrostatic potentials of the protein atoms [17] , [18] . Within the DOCK programme suite, the programme DOCK matches spheres (generated by sphgen_cpp) with small-molecule atoms and uses scoring grids (from grid) to evaluate small-molecule orientations [16] , [17] . DOCK also minimizes energy-based scores. We analysed the 3D solution structure of Bax protein (PDB ID: 1F16) using the UCSF-DOCK 6.0 programme suite as previously described [13] , [19] . Intriguingly, we observed a promising structural pocket around the S184 residue in Bax protein that could be an ideal target for small-molecule docking. This pocket allows us to manipulate the proapoptotic function of Bax as a new anticancer treatment strategy. Here we report the identification of three compounds named small-molecule Bax agonists (that is, SMBA1, SMBA2 and SMBA3) that target S184 site of Bax, activate the proapoptotic function of Bax and potently repress lung tumour growth via induction of apoptosis. These compounds hold potential as an entirely new class of anticancer drugs for the treatment of cancers expressing Bax, including lung cancer. Effect of SMBAs that target S184 site of Bax on apoptosis Phosphorylation or dephosphorylation of Bax at the S184 site negatively or positively regulates the proapoptotic function of Bax [2] , [3] , [9] , suggesting that the S184 site is an attractive target for structure-based drug screening ( Supplementary Fig. 1a ). Approximately 300,000 small molecules from the National Cancer Institute (NCI) database were docked into a structural pocket identified by the DOCK programme suite, which is in close proximity to the S184 residue of Bax protein. After computational screening, 36 small compounds were found to bind to the S184 site of Bax with priority scores ( Supplementary Fig. 1b ). Lung cancer cells express significantly higher levels of endogenous Bax than normal small airway epithelial cells (SAEC) ( Supplementary Fig. 1c ), which suggests that Bax may be a good therapeutic target in human lung cancer. To test whether the 36 small molecules that target Bax at the S184 site induce apoptosis, H1299, A549 and SAEC cells were treated with the molecules (5 μM) for 48 h. Compounds 17, 19 and 20 clearly displayed potent apoptotic effects on human lung cancer H1299 and A549 cells when compared with the other tested small molecules ( Supplementary Fig. 1d ). We named these compounds SMBAs (that is, SMBAs: 17 (NSC408730)→SMBA1 (MW 315), 19 (NSC4436)→SMBA2 (MW 168), 20 (NSC5062)→SMBA3 (MW 308)). Importantly, SMBA1, SMBA2 and SMBA3 induced significantly less apoptosis in normal SAECs that express relatively low levels of Bax compared with H1299 or A549 lung cancer cells ( Supplementary Fig. 1c,d ), indicating their relative selectivity against lung cancer cells. The lead compounds SMBA1, SMBA2 and SMBA3 were also rescored using a molecular dynamics simulation with the all-atom AMBER force field implemented in DOCK 6.5, which is intended for re-scoring existing poses. The resulting AMBER scores showed favourable binding energies for all three compounds (SMBA1: −35.271080, SMBA2: −37.783943 and SMBA3: −14.357678). To test whether the sensitivity of lung cancer cells to SMBA is associated with the phosphorylation status of Bax and/or the total cellular levels of Bax, expression levels of pBax (S184) and Bax in a panel of human lung cancer lines and their sensitivities to the lead compound SMBA1 were analysed by western blot and colony formation, respectively. Levels of pBax from western blot bands were further quantified by ImageJ software as described [20] . Results indicate that human lung cancer cells expressing higher levels of pBax and/or total Bax (that is, H292 and H1975) were more sensitive to SMBA1 at 5 μM ( Supplementary Fig. 2 ). In contrast, human lung cancer H460 cells expressing relatively lower levels of pBax and total Bax were less sensitive to SMBA1 ( Supplementary Fig. 2 ). Interestingly, it seems that human lung cancer cells expressing higher levels of total Bax also contain relatively higher levels of pBax (that is, H292 and H1975) ( Supplementary Fig. 2 ). Based on our findings, we propose that the cytotoxicity of SMBA may be dependent on expression levels of pBax and/or total Bax in human lung cancer cells. To test whether individual SMBA compounds form self-aggregates under the experimental conditions, a dynamic light scattering aggregation assay was performed using increasing concentrations (1, 5, 10, 50, 100, 250 and 500 μM) of SMBA1, SMBA2 and SMBA3. Erlotinib, a drug commonly used to treat lung cancer [21] , was used for comparison. Intriguingly, no self-aggregation of SMBA1, SMBA2 or SMBA3 was observed at concentrations between 1 and 250 μM ( Supplementary Fig. 3 ). For erlotinib, no self-aggregation was observed at concentrations lower than 100 μM ( Supplementary Fig. 3 ). Because the concentrations of SMBA1, SMBA2 or SMBA3 used to measure cytotoxicity in various lung cancer cells were 50 times lower than 250 μM, we can therefore exclude any pseudo-activity caused by aggregates in our system. SMBA(s) binds to Bax and enhances apoptosis of cancer cells Computational modelling analysis reveals that SMBA1, SMBA2 and SMBA3 are small molecules that dock at the S184 binding pocket of Bax ( Fig. 1a ). It has been demonstrated that Bax can heterodimerize with Bak via their BH3 domains to form Bax/Bak heterodimers [22] . The fluorescent Bak BH3 domain peptide (FAM-GQVGRQLAIIGDDINR) is able to bind to the Bax protein with high affinity, thus SMBA(s) may compete with fluorescent Bak BH3 peptide for binding to Bax protein. We used the fluorescent Bak BH3 peptide to measure SMBA/Bax binding affinity in a competition fluorescence polarization assay as described [23] , [24] , [25] . Results indicate that SMBAs selectively bind to Bax protein with high affinities (SMBA1: K i =43.3±3.25 nM, SMBA2: K i =57.2±7.29 nM and SMBA3: K i =54.1±9.77 nM) but fail to bind other Bcl2 family members, including Bcl2, Bcl-XL, Mcl-1, Bcl-w, Bfl-1/A1, Bid or Bak ( Fig. 1b ), indicating the specificity of their Bax binding. These findings suggest that SMBA compounds may be used preferably in those tumours that express elevated levels of Bax. 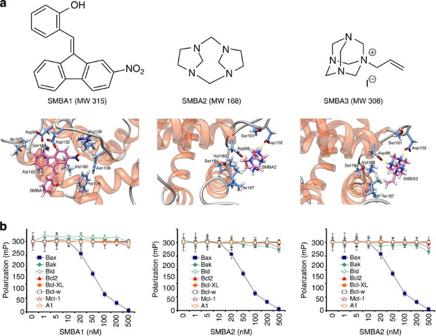Figure 1: SMBA1–3 directly bind to the Bax protein but not to other Bcl2 family members. (a) Structural modelling of SMBA1–3 in the S184 binding pocket in the C terminus of Bax protein using the all-atom AMBER molecular mechanics force field. The PDB files of the modelled complex structures are shown by detailed all-atom views of the predicted interactions for all three compounds along with labels for each residue. (b) Fluorescent Bak BH3 domain peptide (3 nM) was incubated with purified 6 nM of human Bax protein or other Bcl2 family member(s) in the absence or presence of increasing concentrations (that is, 0–500 nM) of SMBA1, SMBA2 or SMBA3 in the binding affinity assay buffer. Binding affinities were analysed using a competition fluorescence polarization assay. The error bars indicate ±s.d. of three separate experiments. Figure 1: SMBA1–3 directly bind to the Bax protein but not to other Bcl2 family members. ( a ) Structural modelling of SMBA1–3 in the S184 binding pocket in the C terminus of Bax protein using the all-atom AMBER molecular mechanics force field. The PDB files of the modelled complex structures are shown by detailed all-atom views of the predicted interactions for all three compounds along with labels for each residue. ( b ) Fluorescent Bak BH3 domain peptide (3 nM) was incubated with purified 6 nM of human Bax protein or other Bcl2 family member(s) in the absence or presence of increasing concentrations (that is, 0–500 nM) of SMBA1, SMBA2 or SMBA3 in the binding affinity assay buffer. Binding affinities were analysed using a competition fluorescence polarization assay. The error bars indicate ±s.d. of three separate experiments. Full size image Our previous findings demonstrated that nicotine can induce Bax phosphorylation at the S184 site [2] . Since SMBAs bind Bax at its S184 phosphorylation site, SMBAs may inhibit nicotine-induced Bax phosphorylation. To test this, A549 cells were metabolically labelled with 32 P-orthophosphoric acid and treated with nicotine in the absence or presence of SMBA1, SMBA2 or SMBA3 (5 μM) for 60 min. Results indicate that treatment of cells with SMBA1, SMBA2 or SMBA3 significantly suppresses nicotine-induced Bax phosphorylation ( Fig. 2a ). Functionally, nicotine can prolong survival of A549 cells following treatment with the therapeutic drug cisplatin, and this effect was abrogated after treatment with SMBA1, SMBA2 or SMBA3 ( Fig. 2b ). Furthermore, the combination of SMBA and cisplatin additively induced apoptosis of human lung cancer cells ( Fig. 2b ). 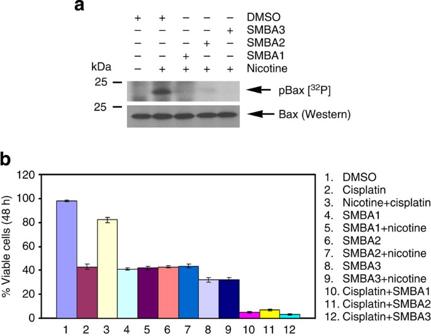Figure 2: SMBAs block Bax phosphorylation and enhance apoptosis. (a) A549 cells were metabolically labelled with [32P]orthophosphoric acid and treated with nicotine (1 μM) in the absence or presence of 5 μM of SMBA1, SMBA2 or SMBA3 for 60 min. Bax phosphorylation was determined by autoradiography (full blots can be found inSupplementary Fig. 6). (b) A549 cells were treated with cisplatin (40 μM), SMBA(s) (5 μM) or in combination in the absence or presence of nicotine (1 μM) for 48 h. Cell viability was analysed by PI-Annexin-V staining with FACS analysis. The error bars indicate ±s.d. of three separate experiments. Figure 2: SMBAs block Bax phosphorylation and enhance apoptosis. ( a ) A549 cells were metabolically labelled with [ 32 P]orthophosphoric acid and treated with nicotine (1 μM) in the absence or presence of 5 μM of SMBA1, SMBA2 or SMBA3 for 60 min. Bax phosphorylation was determined by autoradiography (full blots can be found in Supplementary Fig. 6 ). ( b ) A549 cells were treated with cisplatin (40 μM), SMBA(s) (5 μM) or in combination in the absence or presence of nicotine (1 μM) for 48 h. Cell viability was analysed by PI-Annexin-V staining with FACS analysis. The error bars indicate ±s.d. of three separate experiments. Full size image SMBAs induce Bax mitochondrial insertion and cyt c release Bax is predominantly a cytosolic protein with only a small portion associated with the outer mitochondrial membranes in unstimulated cells [4] . In contrast, cytochrome (Cyt) c is normally localized in mitochondria and can be released into the cytosol following cellular stress [4] . To test whether SMBA-induced inhibition of Bax phosphorylation promotes mitochondrial localization of Bax to initiate Cyt c release, A549 cells were treated with increasing concentrations of SMBA1, SMBA2 or SMBA3 for 24 h. Bax and Cyt c were measured by immunofluorescence. In control cells, Bax displayed a diffuse localization in the cytoplasm while Cyt c exhibited a mitochondrial distribution as punctate staining ( Fig. 3a ). After SMBA treatment, Bax was visible as punctate mitochondrial staining while Cyt c became partially diffuse ( Fig. 3a ). These data suggest that SMBA 1, SMBA2 and SMBA3 facilitate Bax translocation to mitochondria and subsequently induce Cyt c release from mitochondria into the cytosol. It has been demonstrated that an alkali extraction approach can distinguish whether Bax protein only weakly associates with or is directly inserted into mitochondrial membranes [4] , [26] . This approach was used to test whether SMBA can promote Bax insertion into mitochondrial membranes. A549 cells were treated with increasing concentrations of SMBA(s) for 24 h. Mitochondria were isolated, incubated in 0.1 m Na 2 CO 3 , pH 11.5, on ice for 30 min, and centrifuged at 200,000 g to yield a mitochondrial pellet. The resulting alkali-extracted mitochondrial membrane pellet was resuspended in 1% Nonidet P-40 lysis buffer. The alkali-resistant, integral Bax was analysed by western blot. Results reveal that treatment of cells with SMBA enhances Bax insertion into mitochondrial membranes in a dose-dependent manner ( Fig. 3b ). Prohibitin, an integral mitochondrial protein [27] , was not affected by this treatment ( Fig. 3b ). These data suggest that SMBA binding to S184 site promotes Bax insertion into mitochondrial membranes. Subcellular fractionation analysis provided additional evidence that treatment of cells with SMBA1, SMBA2 and SMBA3 promotes Cyt c release ( Fig. 3c ). 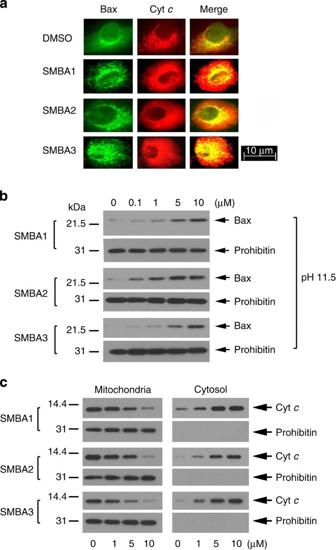Figure 3: SMBAs induce Bax insertion into mitochondrial membranes and Cytcrelease. (a) A549 cells were treated with 5 μM of SMBA1, SMBA2 or SMBA3 for 24 h. Bax and Cytcwere analysed by immunofluorescence staining. Images were merged using Openlab 3.1.5 software. Areas of co-localization are yellow. Scale bar, 10 μm. (b) A549 cells were treated with increasing concentrations of SMBA1, SMBA2 or SMBA3 for 24 h. Mitochondria were isolated and alkali extraction of Bax was performed. The alkali-resistant (that is, non-extractable) Bax was determined by western blot using a Bax antibody (1:500 dilution). (c) A549 cells were treated with increasing concentrations of SMBA1, SMBA2 or SMBA3 for 24 h. Mitochondrial and cytosolic fractions were isolated. Levels of Cytcin these two fractions were analysed by western blot (full blots can be found inSupplementary Fig. 7). Figure 3: SMBAs induce Bax insertion into mitochondrial membranes and Cyt c release. ( a ) A549 cells were treated with 5 μM of SMBA1, SMBA2 or SMBA3 for 24 h. Bax and Cyt c were analysed by immunofluorescence staining. Images were merged using Openlab 3.1.5 software. Areas of co-localization are yellow. Scale bar, 10 μm. ( b ) A549 cells were treated with increasing concentrations of SMBA1, SMBA2 or SMBA3 for 24 h. Mitochondria were isolated and alkali extraction of Bax was performed. The alkali-resistant (that is, non-extractable) Bax was determined by western blot using a Bax antibody (1:500 dilution). ( c ) A549 cells were treated with increasing concentrations of SMBA1, SMBA2 or SMBA3 for 24 h. Mitochondrial and cytosolic fractions were isolated. Levels of Cyt c in these two fractions were analysed by western blot (full blots can be found in Supplementary Fig. 7 ). Full size image Bax is a required target for SMBA induction of apoptosis To test whether Bax is essential for SMBA induction of apoptosis, wild type (WT), Bax −/− , Bak −/− or Bax/Bak double-knockout (DKO) mouse embryonic fibroblasts (MEF) cells were treated with a high concentration of SMBA 1, SMBA2 or SMBA3 (that is, 25 μM) for 24 h. Apoptotic cells were stained with Annexin-V and propidium iodide (PI) and quantified by fluorescence activated cell sorting (FACS) as described previously [28] . Compared with WT and Bak −/− MEF cells, Bax −/− and DKO MEF cells exhibited significant resistance to SMBA1, SMBA2 and SMBA3 ( Fig. 4a,b ). These findings indicate that Bax, but not Bak, is a selective target through which SMBA induces apoptosis. 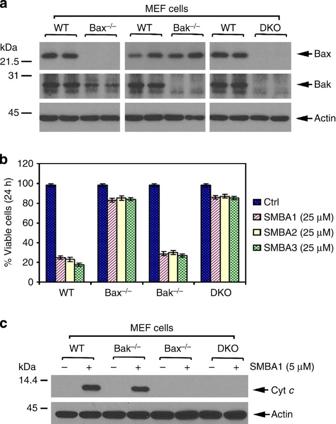Figure 4: Bax is an essential for SMBA induction of apoptosis and Cytcrelease. (a) Levels of Bax were analysed by western blot in wild-type (WT), Bax−/−, Bak−/−or Bax/Bak double-knockout (DKO) MEF cells. (b) WT, Bax−/−, Bak−/−or DKO MEF cells were treated with high concentration (25 μM) of SMBA1, SMBA2 or SMBA3 for 24 h. Cell viability was analysed by PI-Annexin-V staining with FACS analysis. The error bars indicate±s.d. of three separate experiments. (c) Mitochondria were isolated from WT, Bax−/−, Bak−/−or DKO MEF cells. The isolated mitochondria were then treated with lead compound SMBA1 (5 μM) in mitochondrial buffer for 30 min at 30 °C. After centrifugation, Cytcin supernatant fraction (that is, Cytcrelease) and actin in mitochondrial fraction were analysed by western blot (full blots can be found inSupplementary Fig. 8). Ctrl, control. Figure 4: Bax is an essential for SMBA induction of apoptosis and Cyt c release. ( a ) Levels of Bax were analysed by western blot in wild-type (WT), Bax −/− , Bak −/− or Bax/Bak double-knockout (DKO) MEF cells. ( b ) WT, Bax −/− , Bak −/− or DKO MEF cells were treated with high concentration (25 μM) of SMBA1, SMBA2 or SMBA3 for 24 h. Cell viability was analysed by PI-Annexin-V staining with FACS analysis. The error bars indicate±s.d. of three separate experiments. ( c ) Mitochondria were isolated from WT, Bax −/− , Bak −/− or DKO MEF cells. The isolated mitochondria were then treated with lead compound SMBA1 (5 μM) in mitochondrial buffer for 30 min at 30 °C. After centrifugation, Cyt c in supernatant fraction (that is, Cyt c release) and actin in mitochondrial fraction were analysed by western blot (full blots can be found in Supplementary Fig. 8 ). Ctrl, control. Full size image Bax or Bak induces apoptosis by regulating permeability of the mitochondrial outer membrane and escape of apoptogenic factors such as Cyt c [29] . To further test whether SMBA induces Cyt c release from mitochondria in a Bax- but not Bak-dependent fashion, mitochondria were isolated from WT, Bax −/− , Bak −/− or DKO MEF cells. The isolated mitochondria were treated with the lead compound SMBA1 (5 μM) for 30 min at 30 °C. After centrifugation at 13000 g for 5 min, Cyt c in the supernatant (that is, Cyt c release) was analysed by western blot. Results show that SMBA1 induced Cyt c release from the mitochondria isolated from WT and Bak −/− MEF cells but not from Bax −/− or DKO MEF cells, indicating that SMBA1 induces Cyt c release in a Bax- but not Bak-dependent fashion ( Fig. 4c ). SMBAs induce Bax oligomerization in mitochondria To test whether SMBAs affect the conformational change in Bax, we used the 6A7 monoclonal Bax antibody that can specifically detect the Bax conformational change [14] . The antibody 6A7, raised against a peptide comprising amino acids 13–19 of the Bax N terminus, is not able to bind the soluble form of Bax in healthy cells but can recognize Bax after the conformational change associated with membrane insertion that occurs in apoptotic cells [30] , [31] . Recent studies demonstrate that the 6A7 Bax antibody only recognizes conformationally changed, active Bax [3] , [32] . 6A7 antibody binding to Bax was measured by immunofluorescence. Cells were treated with SMBA 1, SMBA2 or SMBA3 (5 μM) for 24 h, and incubated with prewarmed (37 °C) growth medium containing MitoTracker for 30 min. Fixed cells were blocked with 10% mouse serum and then immunostained with the mouse monoclonal 6A7 primary and fluorescein isothiocyanate (FITC)-conjugated anti-mouse secondary antibodies. Although the 6A7 Bax immunofluorescence was low or undetectable in untreated cells, it increased significantly in cells treated with SMBA 1, SMBA2 or SMBA3 ( Fig. 5a ). An immunoprecipitation experiment using 6A7 antibody revealed that SMBAs enhance the ability of Bax to bind to 6A7 antibody ( Fig. 5b ). A similar immunoprecipitation experiment using 6A7 antibody was also performed following incubation of purified Bax protein with SMBA(s) in a cell-free system. Results reveal that SMBA(s) can directly induce Bax conformational change in vitro ( Supplementary Fig. 4 ). These findings suggest that SMBA binding to the S184 site may cause a conformational change that activates the proapoptotic function of Bax. To assess whether SMBAs affect the ability of membrane-inserted Bax to form oligomers in the mitochondrial membrane, a crosslinking study with Bis (maleimido) hexane (BMH) was carried out for measurement of Bax oligomerization. Intriguingly, treatment of A549 cells with SMBA1, SMBA2 or SMBA3 (5 μM) facilitated the formation of Bax dimers and trimers ( Fig. 5c ). The molecular sizes of these adducts were estimated to be multiples of ~21 kDa, suggesting the formation of Bax homo-oligomers in A549 cells. 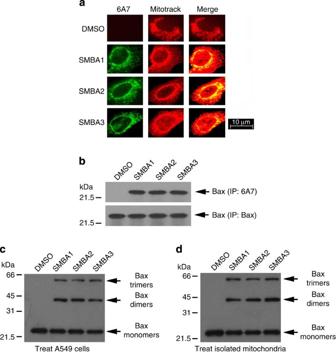Figure 5: SMBA(s) induces Bax conformational change and promotes its oligomerization. (a) A549 cells were treated with 5 μM of SMBA1, SMBA2 or SMBA3 for 24 h. Cells were incubated with prewarmed (37 °C) growth medium containing MitoTracker (red) for 30 min. Cells were then washed with 1 × PBS, fixed, permeabilized with ice-cold methanol and acetone, blocked with 10% mouse serum and stained with mouse monoclonal 6A7 primary and FITC-conjugated anti-mouse secondary (green) antibodies. Images were merged using Openlab 3.1.5 software. Areas of co-localization are yellow. Scale bar, 10 μm. (b) A549 cells were treated with 5 μM of SMBA1, SMBA2 or SMBA3 for 24 h. A co-immunoprecipitation experiment was carried out using the 6A7 or full-length Bax antibody. Bax was analysed by western blot. (c) A549 cells were treated with SMBA1, SMBA2 or SMBA3 (5 μM) for 24 h. After treatment, mitochondria were isolated, followed by crosslinking using BMH. Bax was analysed by western blot. (d) First, mitochondria were isolated from A549 cells and then treated with SMBA1, SMBA2 or SMBA3 (5 μM) in crosslinking buffer for 30 min at 30 °C, followed by crosslinking using BMH. Bax was analysed by western blot (full blots can be found inSupplementary Fig. 9). Figure 5: SMBA(s) induces Bax conformational change and promotes its oligomerization. ( a ) A549 cells were treated with 5 μM of SMBA1, SMBA2 or SMBA3 for 24 h. Cells were incubated with prewarmed (37 °C) growth medium containing MitoTracker (red) for 30 min. Cells were then washed with 1 × PBS, fixed, permeabilized with ice-cold methanol and acetone, blocked with 10% mouse serum and stained with mouse monoclonal 6A7 primary and FITC-conjugated anti-mouse secondary (green) antibodies. Images were merged using Openlab 3.1.5 software. Areas of co-localization are yellow. Scale bar, 10 μm. ( b ) A549 cells were treated with 5 μM of SMBA1, SMBA2 or SMBA3 for 24 h. A co-immunoprecipitation experiment was carried out using the 6A7 or full-length Bax antibody. Bax was analysed by western blot. ( c ) A549 cells were treated with SMBA1, SMBA2 or SMBA3 (5 μM) for 24 h. After treatment, mitochondria were isolated, followed by crosslinking using BMH. Bax was analysed by western blot. ( d ) First, mitochondria were isolated from A549 cells and then treated with SMBA1, SMBA2 or SMBA3 (5 μM) in crosslinking buffer for 30 min at 30 °C, followed by crosslinking using BMH. Bax was analysed by western blot (full blots can be found in Supplementary Fig. 9 ). Full size image To further test whether SMBAs directly activate Bax through formation of oligomers in the isolated mitochondria, crosslinking studies with BHM were used following direct treatment of the isolated mitochondria with SMBA1, SMBA2 or SMBA3 as described [22] , [33] . Results indicate that direct treatment of isolated mitochondria with SMBA1, SMBA2 or SMBA3 resulted in formation of Bax dimers and trimers in mitochondria ( Fig. 5d ). The pattern of Bax oligomers is similar to that in the treated cells as above. These findings provide direct evidence that SMBAs can activate Bax through its oligomerization in isolated mitochondrial membranes. SMBA1 suppresses tumour growth via apoptosis in vivo To test the in vivo efficacy of SMBA, we used nude mice to produce subcutaneous lung tumour xenografts as described [34] , [35] . Treatment of mice with increasing doses (that is, 2–60 mg kg −1 ) of SMBA1 resulted in a dose-dependent repression of lung cancer in vivo ( Fig. 6a ). Since similar potency was observed in mice treated with 40 and 60 mg kg −1 , this suggests that 40 mg kg −1 may be a suitable dose for suppression of lung cancer growth in xenograft models. To test whether SMBA1-induced suppression of lung cancer occurs through apoptosis in lung tumour tissues, active caspase 3 was measured by immunohistochemistry (IHC). Intriguingly, treatment of lung cancer xenograft mice with SMBA1 resulted in increased levels of active caspase 3 ( Fig. 6b ). No weight loss, no significant increase in alanine aminotransferase (ALT), aspartate aminotransferase (AST) and blood urea nitrogen (BUN) or decrease in white blood cells (WBC), red blood cells (RBC), haemoglobin (Hb) and platelets (PLT) were observed following SMBA1 treatment ( Fig. 7a,b ). Histopathology of harvested normal tissues (brain, heart, lung, liver, spleen, kidney and intestine) revealed no evidence of normal tissue toxicity ( Fig. 7c ). 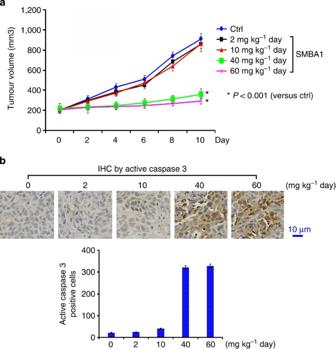Figure 6: SMBA suppresses lung cancerin vivo. (a) Nu/Nu mice with A549 lung cancer xenografts were treated with increasing doses of SMBA1 (2~60 mg kg−1per day) intraperitoneally for 10 days. Each group includes eight mice. Tumour volume was measured once every 2 days. The error bars indicate ±s.d. Statistical significance was analysed with two-sided unpaired Student’st-test. After 10 days, the mice were sacrificed and the tumours were removed and analysed. (b) Active caspase 3 was analysed in tumour tissues at the end of experiments by IHC staining. Scale bar, 10 μm. The error bars indicate ±s.d. Ctrl, control. Figure 6: SMBA suppresses lung cancer in vivo . ( a ) Nu/Nu mice with A549 lung cancer xenografts were treated with increasing doses of SMBA1 (2~60 mg kg −1 per day) intraperitoneally for 10 days. Each group includes eight mice. Tumour volume was measured once every 2 days. The error bars indicate ±s.d. Statistical significance was analysed with two-sided unpaired Student’s t -test. After 10 days, the mice were sacrificed and the tumours were removed and analysed. ( b ) Active caspase 3 was analysed in tumour tissues at the end of experiments by IHC staining. Scale bar, 10 μm. The error bars indicate ±s.d. Ctrl, control. 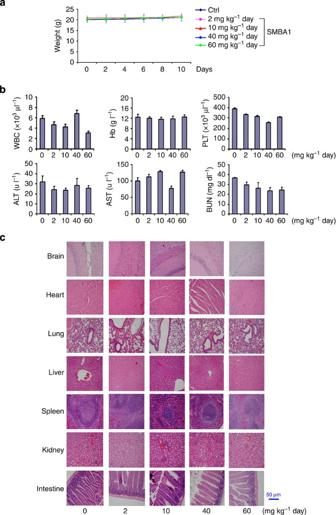Figure 7: Analysis of SMBA toxicityin vivo. (a) Body weight of mice was measured once every other day during treatment with increasing doses of SMBA1 (2–60 mg kg−1per day). The error bars indicate ±s.d. (b) Blood analysis of mice after treatment with SMBA1. The error bars indicate ±s.d. (c) Haematoxylin and eosin histology of various organs from mice after treatment with SMBA1. Scale bar, 50 μm. Ctrl, control; Hb, haemoglobin; WBC, white blood cell. Full size image Figure 7: Analysis of SMBA toxicity in vivo . ( a ) Body weight of mice was measured once every other day during treatment with increasing doses of SMBA1 (2–60 mg kg −1 per day). The error bars indicate ±s.d. ( b ) Blood analysis of mice after treatment with SMBA1. The error bars indicate ±s.d. ( c ) Haematoxylin and eosin histology of various organs from mice after treatment with SMBA1. Scale bar, 50 μm. Ctrl, control; Hb, haemoglobin; WBC, white blood cell. Full size image QD-IHF analysis of pBax and 6A7 Bax in tumour tissues The quantum dot-immunohistofluorescence (QD-IHF) technique is a valuable tool for simultaneous and concurrent detection of multiple biomarkers in formalin-fixed paraffin-embedded tissues, thereby allowing for quantification of several biomarkers simultaneously on the same tissue slide [36] , [37] , [38] , [39] . To confirm whether SMBA can convert Bax from its inactive (pS184 Bax) to active form (6A7 Bax), pBax and 6A7 Bax were simultaneously analysed by QD-IHF on the same tissue slide using primary antibodies from different sources (that is, pBax antibody from rabbit and 6A7 antibody from mouse) and QD-conjugated anti-rabbit (that is, QD605 (red)) and anti-mouse (that is, QD705 (green)) secondary antibodies with two different emission wavelengths. Both separated and combined QD images were obtained after determining the QD spectral library and unmixing the cubed image. Intriguingly, treatment of A549 xenograft mice with SMBA1 (40 mg kg −1 per day) for 10 days resulted in decreased Bax phosphorylation (that is, pS184 Bax) and increased Bax conformational change (that is, 6A7 Bax) in tumour tissues ( Supplementary Fig. 5 ). These findings suggest that treatment of mice with SMBA may induce the conversion of inactive Bax to the activated form and eventually lead to apoptosis in tumour tissues. Bax is required for SMBA to repress lung cancer in vivo We have previously established lung cancer A549 cells in which Bax was stably depleted by RNA interference using a vector-based gene silencing approach [2] , [40] . The pSilencer 2.1-U6 hygromycin plasmids bearing the Bax hairpin siRNA insert were transfected into A549 cells. The stable clones persistently produce Bax siRNA to interfere with Bax expression in A549 cells. A549 cells expressing Bax siRNA displayed >99% reduction of Bax protein expression ( Fig. 8a ). To test whether Bax expression is essential for SMBA’s antitumour activity in vivo , mice bearing lung cancer xenografts derived from A549 cells expressing Bax siRNA or control siRNA were treated with SMBA1 (40 mg kg −1 per day) for 14 days. Results indicate that lung cancer xenografts derived from control A549 cells were sensitive to SMBA1, while xenografts derived from A549 cells expressing Bax siRNA were resistant ( Fig. 8b ). Intriguingly, increased active caspase 3 was observed in the control xenografts but not in the Bax siRNA-xenografts ( Fig. 8c ). These findings suggest that Bax expression is essential for SMBA1 suppression of lung cancer in vivo . 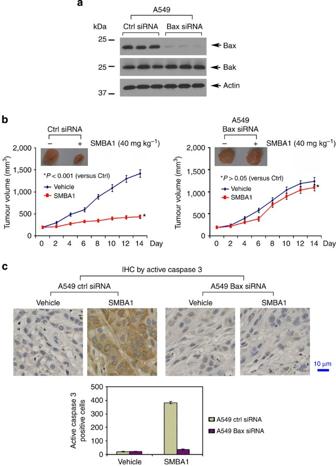Figure 8: Bax is essential for SMBA suppression of lung cancer in xenograft models. (a) Expression levels of Bax and Bak in A549 cells that persistently express Bax siRNA or control (Ctrl) siRNA were analysed by western blot (full blots can be found inSupplementary Fig. 10). (b,c) Mice with xenografts derived from A549 expressing Bax siRNA, or Ctrl siRNA were treated with SMBA1 (40 mg kg−1) or vehicle for 14 days. Tumour volume and active caspase 3 in tumour tissues were analysed. Scale bar, 10 μm. The error bars indicate ±s.d. Statistical significance was analysed with two-sided unpaired Student’st-test. Figure 8: Bax is essential for SMBA suppression of lung cancer in xenograft models. ( a ) Expression levels of Bax and Bak in A549 cells that persistently express Bax siRNA or control (Ctrl) siRNA were analysed by western blot (full blots can be found in Supplementary Fig. 10 ). ( b , c ) Mice with xenografts derived from A549 expressing Bax siRNA, or Ctrl siRNA were treated with SMBA1 (40 mg kg −1 ) or vehicle for 14 days. Tumour volume and active caspase 3 in tumour tissues were analysed. Scale bar, 10 μm. The error bars indicate ±s.d. Statistical significance was analysed with two-sided unpaired Student’s t -test. Full size image Survival outcomes remain poor for lung cancer patients in large part owing to resistance to conventional therapeutic interventions [41] . Apoptotic induction in cancer cells is an established paradigm in cancer therapy. Bax has been identified as a promising prognostic indicator in patients with lung cancer [42] , suggesting that it could potentially also offer a therapeutic target in lung cancer patients. We recently identified that the S184 phosphorylation site in the C-terminal tail of Bax functionally controls the proapoptotic activity of Bax [2] , [3] . Here we chose the S184 residue as a docking site for screening of small molecules and identified three compounds (that is, SMBA1–3) that induce greater apoptosis in lung cancer cells than in normal cells ( Supplementary Fig. 1 ). Using a competition fluorescence polarization assay, we found that all three SMBA compounds directly and tightly bind to purified Bax protein but not to other Bcl2 family members in vitro ( Fig. 1b ), indicating a selective Bax binding. Treatment of lung cancer cells with SMBA1, SMBA2 or SMBA3 inhibits Bax phosphorylation and promotes apoptosis of lung cancer cells ( Fig. 2 ), suggesting that SMBAs may target the Bax phosphorylation site in cells. Bax is found in both the cytosolic and mitochondrial fractions in many cultured cells [4] , [30] , [43] . Alkali extraction studies in vitro have further demonstrated that most Bax is lost from mitochondrial membranes during this treatment, indicating that under normal conditions Bax is loosely attached to mitochondria [4] , [26] , [44] . SMBAs promote the ‘peripherally’ associated mitochondrial Bax to insert into mitochondrial membranes leading to Bax membrane integration and Cyt c release ( Fig. 3 ). The lead compound SMBA1 stimulates Cyt c release from mitochondria in a Bax- but not Bak-dependent fashion. Furthermore, Bax −/− and DKO MEF cells were significantly resistant to SMBAs at a high concentration (25 μM), whereas WT and Bak −/− MEF cells were relatively sensitive ( Fig. 4 ). Based on these findings, we propose that Bax, but not Bak, is a required target for SMBA-induced apoptosis. Treatment of human lung cancer A549 cells with SMBA results in a conformational change detected by the 6A7 Bax antibody, which only recognizes active, conformationally changed Bax ( Fig. 5a,b ), suggesting that the binding of SMBA with Bax may result in exposure of the 6A7 epitope, which is normally hidden in its N terminus. Immunofluorescence analysis using the 6A7 Bax antibody following treatment of cells with SMBA(s) exhibits punctate staining of Bax localized within mitochondria ( Fig. 5a ), indicating that the 6A7 epitope-specific conformational change resulting from SMBA/Bax binding enables Bax to bind to mitochondria. Using a chemical crosslinker approach, we found that treatment of either cells or isolated mitochondria with SMBA(s) facilitates the formation of Bax oligomers, including dimers and trimers ( Fig. 5c,d ). It has been demonstrated that Bax oligomers can form a pore size that is capable of transporting Cyt c [45] . In support of this, our findings indicate that SMBA-stimulated Bax oligomerization is associated with increased Cyt c release ( Figs 3 and 5 ). It is possible that the SMBA-activated Bax molecules may more efficiently form large structures (that is, oligomers) in mitochondrial membranes to allow the passage of proteins at least of the size of Cyt c . These results reveal a novel mechanism by which SMBA(s) enhances the proapoptotic activity of Bax. Recently, a small molecule (BAM7) has been discovered to specifically activate Bax by targeting Bax at its trigger site [46] . Clearly, the mechanisms by which BAM7 and SMBA activate Bax are different. It remains unclear whether BAM7 has antitumour activity in vivo . We also evaluated the antitumour activity of SMBA in lung cancer xenografts. The lead compound SMBA1 potently represses lung cancer in association with increased apoptosis in tumour tissues ( Fig. 6 ). Intriguingly, SMBA1 has no significant effect in Bax-deficient lung cancer xenografts ( Fig. 8 ), indicating that Bax expression in the tumour is essential for SMBA suppression of tumour growth in vivo . Since no significant normal tissue toxicity in vivo was observed at the effective dose ( Fig. 7 ), this suggests that SMBA(s) may have great potential to be developed as a new class of anticancer drug(s). QD-based images showed that Bax activator SMBA1 can reduce levels of the inactive form of Bax (pS184 Bax) and enhance the activated form of Bax (that is, 6A7 conformationally changed Bax) in tumour tissues ( Supplementary Fig. 5 ). Based on findings from lung cancer xenografts and QD-IHF analysis, we propose that SMBA-induced suppression of lung cancer may result from selective activation of the proapoptotic function of Bax leading to increased apoptosis in tumours. Significant effort has been devoted to targeting the native form of Bcl2 protein in solid malignancies and in haematological cancers. However, clinical trials of Bcl2-targeted agents (that is, ABT-737, ABT-263 and so on) have been less successful than was anticipated [47] , [48] . The development of previously unforeseen toxicity, such as thromobocytopenia, compromised efficacious dosing in clinical testing [47] . Our approach to targeting Bax may overcome these challenges because phosphorylated Bax is a biological gatekeeper of the proapoptotic function of this protein. Moreover, the S184 phosphorylation site is not shared with other Bcl2 family members, thereby minimizing the likelihood that SMBAs may affect other Bcl2 protein members with unwanted toxicity. This expectation is substantiated by the lack of normal tissue toxicity in mice treated with the efficacious dose of these agents in our xenograft experiments ( Fig. 7 ). In summary, we have discovered novel Bax activators (SMBA1–3) that specifically target the binding pocket at S184, cause Bax conformational change, and facilitate Bax homo-oligomerization leading to Bax activation and apoptosis in lung cancer cells. The lead compound SMBA1 has potent activity against lung cancer by selectively activating Bax in vivo . Based on our findings showing selective efficacy in lung cancer as proapoptotic agents without evidence of any surrounding normal tissue toxicity, SMBAs potentially represent a novel class of anticancer drugs for the treatment of lung cancer by specifically targeting Bax at the S184 binding pocket in its hydrophobic C-terminal tail. Materials All small molecules utilized were obtained from the NCI ( http://dtp.nci.nih.gov/RequestCompounds ). Nicotine and cisplatin were purchased from Sigma-Aldrich (St Louis, MO, USA). Primary anti-Bax, FITC-conjugated anti-mouse and rhodamine-conjugated anti-rabbit secondary antibodies were purchased from Santa Cruz Biotechnology (Santa Cruz, CA, USA). Bax 6A7 and Cyt c antibodies were obtained from BD Pharmingen (San Diego, CA, USA). The phospho-specific S184 Bax (pBax) antibody was purchased from Abcam (Cambridge, MA, USA). Active caspase 3 antibody was obtained from Cell Signaling Technology (Beverly, MA, USA). Purified recombinant Bax protein was obtained from Novus (Littleton, CO, USA). Protease inhibitor cocktail set I and digitonin were purchased from EMD Millipore (Billerica, MA, USA). BMH was purchased from Thermo Scientific (Rockford, IL, USA). 32 P-orthophosphate was purchased from MP Biomedicals (Irvine, CA, USA). All reagents used were obtained from commercial sources unless otherwise stated. Computational screening of SMBAs In order to identify potential Bax agonists, we used a high throughput in silico molecular docking strategy using UCSF-DOCK 6.0. Our computational screen was directed toward the solution structure of Bax (PDB ID: 1F16; ref. 12 ). We have created a subset of the NCI Developmental Therapeutics Library of ~300,000 small molecules that follow the Lipinski rules for ‘drug-like’ compounds [49] . These small molecules from the NCI/developmental therapeutic program (DTP) database were docked into a structural pocket characterized by the Dock suite programme SPHGEN_CPP, which was in close proximity to residue S184 (that is, a major phosphorylation site of Bax) [2] , [9] , [14] . The receptor structure was prepared using ‘Dock Prep’ function in the UCSF Chimera software [50] . As part of the docking preparations, all water molecules were removed from the solution structure. Any incomplete side chains with missing atoms in the solution structure were replaced using the Dunbrack rotamer library [51] . Hydrogens were added to the entire receptor and hydrogen bonds were identified where possible. Partial charges were calculated for the entire receptor with the AMBER module ANTECHAMBER using the Gasteiger method. The completed receptor was saved in MOL2 format, which is the input to the grid-based scoring function grid from the DOCK 6.0 package. Grid uses this structure to generate the scoring grids for electrostatic and Van der Waals (vDW) interactions with the docked ligands. The docking parameters included testing 1,000 orientations of each input small molecule, followed by energy minimization. Scored compounds were then ranked based on total energy score, consisting of the non-bonded terms of the AMBER molecular mechanics force field. To re-score the existing poses, a molecular dynamics simulation with the all-atom AMBER force field implemented in DOCK 6.5 was also used. Rather than the flexible-ligand/rigid-receptor paradigm common to docking, the AMBER score in DOCK 6.5 allows distance-based receptor flexibility and full-ligand flexibility. This simulation uses the Generalized Born implicit solvation model. The three molecules and the receptor protein were first parameterized using the ‘prepare_amber.pl’ Perl script provided with DOCK 6.5. Hundred cycles of minimization were then performed. Three-thousand steps of Langevin molecular dynamics were performed at a constant temperature of 300 K. Finally, another 100 steps of minimization were performed and the total energy of the complex was evaluated. We allowed all atoms in the receptor molecule within 10 Å of the ligand to move throughout this simulation in order to simulate ‘induced fit’ dynamics. Cell lines and cell culture WT, Bax −/− , Bax/Bak DKO MEF cells were obtained from Dr. Douglas R. Green (St. Jude Children’s Research Hospital, Memphis, TN, USA) and maintained in DMEM medium with 10% fetal bovine serum. Bak −/− MEF cells, normal SAEC and lung cancer cell lines were purchased from the American Type Culture Collection (Manassas, VA, USA). SAEC cells were cultured in small airway epithelial growth media (SAGM BulletKit, American Type Culture Collection). Lung cancer cell lines (that is, H69, H82, H23, H292, H460, H157, H1299, H1975 and Calu-1) were maintained in RPMI 1640 with 10% fetal bovine serum. A549 cells were cultured in F-12K medium with 10% fetal bovine serum. These cell lines were used for the described experiments without further authentication. Mitochondrial isolation and Bax oligomerization assay Digitonin-based mitochondrial isolation and Bax oligomerization analysis was carried out as described [22] , [33] , [52] . Briefly, 3 × 10 7 A549 cells were washed three times with cold 1 × PBS and then incubated with permeabilization buffer (20 mM HEPES/KOH, pH 7.5, 100 mM sucrose, 2.5 mM MgCl 2 , 50 mM KCl and 0.025% digitonin) with protease inhibitor cocktail set I for 5 min on ice. Supernatant and membrane pellet fractions were separated by centrifugation at 13,000 g for 5 min. Membrane fraction was treated with crosslinker BMH (0.5 mM) in crosslinking buffer (20 mM HEPES/KOH, pH 7.0, 100 mM sucrose, 2.5 mM MgCl 2 and 50 mM KCl) for 30–60 min at room temperature. The reaction was quenched by addition of reducing sample buffer, boiled for 5 min and then subjected to SDS-PAGE gels and analysed by western blot using a Bax antibody (1:500 dilution). Lung cancer xenografts and treatments The Institutional Animal Care and Use Committee of Emory University approved the animal experiments. Six-week-old male Nu/Nu nude mice were purchased from Harlan and housed under pathogen-free conditions in microisolator cages. Xenografts were raised by injecting 5 × 10 6 of A549 cells in a balanced salt solution into subcutaneous tissue at the flank region of nude mice. The tumours were allowed to grow to an average volume of 230–250 mm 3 before initiation of therapy as described [34] , [53] . The mice bearing A549 xenografts were treated with vehicle control (that is, 0.5% DMSO) or SMBA1 (2–60 mg kg −1 ) administered intraperitoneally once daily for 10 days. Tumour volume (V) was measured by caliper measurements once every 2 days and calculated with the formula: V=L × W 2 /2 (L, length; W, width) as described [54] . At the end of experiments, mice were euthanized by CO 2 inhalation. Harvested tumour tissues were used for further analysis. Statistical analysis Significant difference between two groups was analysed with two-sided unpaired Student’s t -test. Results were considered to be statistically significant at P <0.05. Statistical analysis was performed with GraphPad InStat 3 software (San Diego, CA, USA) [55] . How to cite this article: Xin, M. et al . Small-molecule Bax agonists for cancer therapy. Nat. Commun. 5:4935 doi: 10.1038/ncomms5935 (2014).